Functional interplay between Aurora B kinase and Ssu72 phosphatase regulates sister chromatid cohesion Cohesins establish cohesion between replicated sister chromatids and are maintained as a multiprotein complex on chromosome arms until they are phosphorylated by mitotic kinases, such as Aurora B and Plk1. However, the mechanics of how the phosphorylation and dephosphorylation of cohesin subunits by kinases and phosphatases, respectively, leads to the dissociation of the cohesin complex from chromosomes remain unclear. Here we report that Aurora B kinase directly interacts with and phosphorylates Ssu72, a new cohesin-binding phosphatase, at Ser 19 in vitro and in vivo . The Aurora B-mediated phosphorylation of Ssu72 causes the structural modification of Ssu72 protein, downregulates phosphatase activity and triggers the ubiquitin-dependent degradation of Ssu72. Overexpression of the Aurora B-mediated phosphomimetic mutant of Ssu72 prevents maintainance chromosome arm cohesion. These results provide evidence that Aurora B kinase directly targets Ssu72 phosphatase for regulation of sister chromatid cohesion during early mitosis. Sister chromatid separation during mitosis depends on the removal of cohesins from chromosomes. This process involves two mechanisms in vertebrate cells [1] : the dissociation of cohesins from chromosome arms in prophase and the proteolytic cleavage of cohesins at centromeres in metaphase. The prophase pathway depends on a process requiring Plk1, Aurora B and Wapl, a cohesin-associated protein [2] , [3] , [4] , [5] , [6] , whereas the metaphase pathway is mediated by separase following its activation by the anaphase-promoting complex/cyclosome [7] . Recent studies have suggested that the phosphorylation of cohesin subunits, such as SA2 and Rad21/Scc1, occurs in a mitosis-specific manner and is required for the stepwise removal of chromosome arm cohesion [1] , [8] . It should also be noted that SA2 phosphorylation by Plk1 and shugoshin (Sgo1) relocation by Aurora B during early mitosis are required for the dissociation of cohesins from the chromosome arm [2] , [4] , [8] . Importantly, the expression of non-phosphorylatable SA2 prevents the removal of chromosome arm cohesion during prophase and prometaphase [8] , indicating that the phosphorylation of this cohesin subunit is indispensable for the dissociation of chromosome cohesin in early mitosis. However, the mechanics of how the phosphorylation of cohesin subunits by mitotic kinases leads to the dissociation of the cohesin complex from chromosomes remain unclear, as is the nature of the protection of the cohesin complex from dissociation before the onset of mitosis. The temporal posttranslational modification (phosphorylation and acetylation) states of the cohesin complex and its regulatory proteins are tightly linked to the proper establishment and stepwise dissociation of sister chromatid cohesion. Protein phosphatase 2A (PP2A) and Sgo1 function together to protect centromeric cohesin during early mitosis [9] , [10] . More specifically, PP2A–Sgo1 complex localizes to the centromere and counteracts the phosphorylation of cohesins by Plk1 and potentially by Aurora B [9] , [11] . Recently, it has been reported that Sgo1 has a PP2A-independent role in the protection of chromosome arm cohesion, because PP2A is unable to localize at the chromosome arm [12] , [13] . Therefore, it is unlikely that PP2A is involved in inhibiting the signalling event of chromosome arm cohesion that is catalysed by these mitotic kinases. The cohesin complex also undergoes acetylation during DNA replication, and this modification is known to be essential for establishing cohesion [14] , [15] , [16] , [17] , [18] . The establishment of cohesion between the sister chromatids is modulated by a number of other cohesin-associated proteins, including Esco1/2 (homologue of acetyltransferase Eco1), Pds5 and Sororin [19] , [20] , [21] . Esco1 and Esco2 can acetylate on K105 and K106 of Smc3 (K112 and K113, respectively, in yeast) [16] , thereby facilitating sororin recruitment to chromatin [22] , [23] . In contrast, Wapl is a negative regulator of cohesion maintenance required for the dissociation of arm cohesin by facilitating the opening of the cohesion ring during early mitosis in vertebrate cells [5] , [6] . Wapl contains several FGF (Phe-Gly-Phe) motifs that regulate the interaction with both Pds5 and Rad21/Scc1 of cohesion subunits [13] , [22] . Another component of the cohesin entourage is sororin [24] . Unlike other cohesin components, sororin is not present in yeast but is essential for cohesion establishment and/or maintenance in eukaryotic cells. Interestingly, sororin also contains an FGF sequence motif that mediates the binding of Pds5 and thus can inhibit the cohesion-destabilizing function of Wapl during the S or G2 phase [22] . Recent studies have shown that sororin is phosphorylated by Cdk1 and Plk1 from entering mitosis and that the mitotic phosphorylation of sororin reduces its ability to inhibit the interaction between Wapl and Pds5, allowing for the resolution of arm cohesins in prophase [25] , [26] , [27] . Collectively, these demonstrate that the periodic posttranslational modifications of cohesin components are tightly connected with the cell cycle progression. Ssu72 has been characterized as an RNA polymerase II carboxy-terminal domain (RNAPII CTD) phosphatase that specifically catalyses serine-5-p dephosphorylation [28] . The amino-acid sequence of Ssu72 includes the CX5RS signature motif of a protein tyrosine phosphatase but possesses a variant ‘aspartate loop’ suggestive of a new class of protein phosphatases [28] , [29] , [30] . Ssu72 can directly interact with Rad21 and SA2, and the depletion or mutational inactivation of the Ssu72 phosphatase can cause the premature separation of the sister chromatid arm [31] . In addition, although Ssu72 counteracts the phosphorylation of SA2, it does not counteract that of other cohesin subunits, and it dephosphorylates SA2 (ref. 31 ). Together, these findings indicate that the Ssu72 phosphatase is capable of maintaining cohesion between sister chromatid arms. In this study, we show that the Aurora B kinase functionally interacts with the Ssu72 phosphatase in regulating sister chromatid cohesion during early mitosis. Our results provide a better understanding of the way in which cohesin maintains chromosome arm cohesion and protects against the premature removal of cohesion in the G2 phase or early mitosis. Ssu72 is required for chromatid cohesion after S-phase To examine the coupling of Ssu72 expression to sister chromatid cohesion during the cell cycle, we used small hairpin RNA (shRNA) to deplete the Ssu72 of HeLa cells. Synchronized cells in G2 phase were pulse labelled with bromodeoxyuridine (BrdU) and then processed for fluorescence in situ hybridization (FISH) using a probe for the arm region on chromosome 21 (Down syndrome critical region 4) to measure the distance between the sister chromatids ( Fig. 1a ). For the assessments of the degree of Ssu72 depletion and the cell cycle profiles of synchronized cells, the synchronized cells were collected, and then immunoblotting and FACS analyses were carried out ( Fig. 1b ). In the control cells, the average distance between paired FISH signals was 0.41 μm in chromosome 21. As predicted, Ssu72 depletion significantly changed the average interchromatid distance between FISH signals: 0.74 μm in chromosome 21 ( Fig. 1c ). We then used another probe for the arm region on chromosome 7 (c-MET). Similarly, the distance between paired FISH signals of Ssu72-depleted cells showed a marked increase (the average distance: 0.69 μm) compared with the control cells (the average distance: 0.39 μm) ( Fig. 1d,e ). These results imply that the Ssu72 function was indeed indispensable in preventing premature cohesin removal in the G2 phase. However, the distance between paired FISH signals in S-phase cells was indistinguishable from that between the control and Ssu72-depleted cells, whereas Rad21 depletion in the S‐phase causes a substantial increase in the distance between FISH signals ( Supplementary Fig. S1 ). This indicates that the function of Ssu72 was required for sister chromatid cohesion after the S-phase. 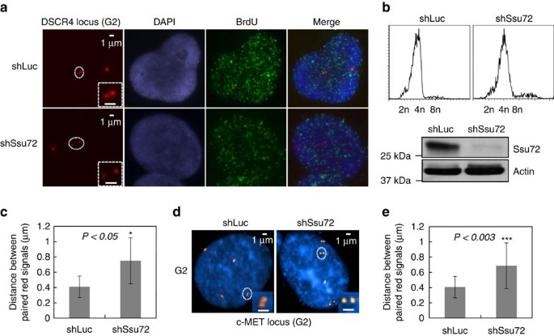Figure 1: Ssu72 is required for sister chromatid cohesion during the G2 phase. (a) HeLa cells were transfected with luciferase (shLuc) or Ssu72 (shSsu72) shRNA and synchronized in G2 phase by the double-thymidine block and release for 6 h; the cells were then incorporated with BrdU for 30 min. Cells were fixed and subjected to FISH with specific probe for the arm locus on chromosome 21 (21q22, Down syndrome critical region 4: DSCR4). BrdU-incorporated nuclei (green) with three pairs of FISH signals (red) are shown. Scale bars represent 1 μm. (b) Synchronized cells were analysed by flow cytometry to determine their DNA content and by immunoblotting with anti-Ssu72 and anti-Actin antibodies. (c) The distance between paired FISH signals was quantified using Huygens software (mean±standard deviation [s.d.]; n≥70 chromosomes were counted per experiment). The asterisk denotes a difference according to Student’st-test (*P<0.05). (d) FISH of specific probe for the arm locus on chromosome 7 (7q31, c-MET). Scale bars represent 1 μm. (e) Quantification of the distance between paired FISH signals inFig. 1d(mean±s.d.; n≥70 chromosomes were counted per experiment, ***P<0.003, Student’st-test). Figure 1: Ssu72 is required for sister chromatid cohesion during the G2 phase. ( a ) HeLa cells were transfected with luciferase (shLuc) or Ssu72 (shSsu72) shRNA and synchronized in G2 phase by the double-thymidine block and release for 6 h; the cells were then incorporated with BrdU for 30 min. Cells were fixed and subjected to FISH with specific probe for the arm locus on chromosome 21 (21q22, Down syndrome critical region 4: DSCR4). BrdU-incorporated nuclei (green) with three pairs of FISH signals (red) are shown. Scale bars represent 1 μm. ( b ) Synchronized cells were analysed by flow cytometry to determine their DNA content and by immunoblotting with anti-Ssu72 and anti-Actin antibodies. ( c ) The distance between paired FISH signals was quantified using Huygens software (mean±standard deviation [s.d. ]; n≥70 chromosomes were counted per experiment). The asterisk denotes a difference according to Student’s t -test (* P <0.05). ( d ) FISH of specific probe for the arm locus on chromosome 7 (7q31, c-MET). Scale bars represent 1 μm. ( e ) Quantification of the distance between paired FISH signals in Fig. 1d (mean±s.d. ; n≥70 chromosomes were counted per experiment, *** P <0.003, Student’s t -test). Full size image Periodic regulation of Ssu72 phosphatase activity The tight coupling of cohesion maintenance to the cell cycle suggests that control of cell cycle progression may be associated with the phosphatase activity and/or function of Ssu72. First, for an analysis of the phosphatase activity of Ssu72 during the cell cycle, HeLa cells were synchronized in the G1-S boundary by the double-thymidine block, in the G2 phase by doxorubicin treatment and in mitosis by nocodazole treatment. Cellular extracts from synchronized cells were processed for immunoprecipitation ( Fig. 2a ), and the phosphatase activity was analysed using the endogenous Ssu72 complex ( Fig. 2b ). The results indicate that the phosphatase activity of Ssu72 was maintained in both the G1/S and G2 phases but declined sharply in cells synchronized in mitosis, implying that the phosphatase activity of Ssu72 was periodically regulated during the cell cycle. In addition, we observed a prematurely hyperphosphorylated form of SA2 in the G2 phase. Interestingly, the levels of hyperphosphorylated SA2 were significantly increased in Ssu72 knockdown cells ( Fig. 2c ). Consistent with a previous report [31] , we were able to detect the SA2 hyperphosphorylaton in the non‐chromatin fractions of G2 and mitotic cellular extracts in the Ssu72‐depleted cells ( Fig. 2d ). These findings therefore indicate that the function of Ssu72 in hyperphosphorylating/dephosphorylating SA2 depends on the periodic regulation of Ssu72’s phosphatase activity during the cell cycle. 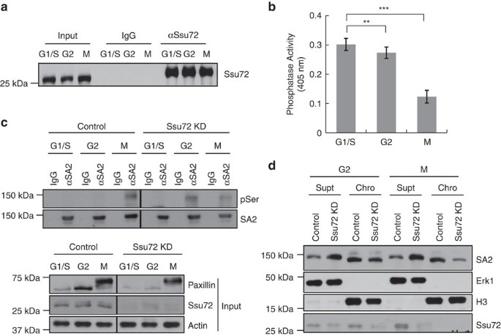Figure 2: Periodic regulation of Ssu72 phosphatase activity during the cell cycle. (a–d) HeLa cells were synchronized in the G1/S boundary by using the double-thymidine block, in the G2 phase by doxorubicin treatment and in mitosis by nocodazole treatment. (a) Cellular extracts from synchronized cells were immunoprecipitated with the anti-Ssu72 antibody and then analysed by immunoblotting. (b) Purified Ssu72 proteins were incubated in a phosphatase buffer containing 10 mM pNPP. **P<0.01 and ***P<0.001, Student’st-test; Error bars represent s.d. values from three independent experiments. (c) Cellular extracts from synchronized Control HeLa and Ssu72 knockdown (Ssu72 KD) cells were immunoprecipitated with normal immunoglobulin G (IgG) or an anti-SA2 antibody and immunoprecipitates were analysed by immunoblotting with anti-phospho-serine and anti-SA2 antibodies. (d) Synchronized cells were separated into non-chromatin supernatant (Supt) and chromatin (Chro) fractions, resolved by SDS–PAGE, and immunoblotted with anti-SA2, anti-Erk1, anti-H3 and anti-Ssu72 antibodies. Figure 2: Periodic regulation of Ssu72 phosphatase activity during the cell cycle. ( a – d ) HeLa cells were synchronized in the G1/S boundary by using the double-thymidine block, in the G2 phase by doxorubicin treatment and in mitosis by nocodazole treatment. ( a ) Cellular extracts from synchronized cells were immunoprecipitated with the anti-Ssu72 antibody and then analysed by immunoblotting. ( b ) Purified Ssu72 proteins were incubated in a phosphatase buffer containing 10 mM pNPP. ** P <0.01 and *** P <0.001, Student’s t -test; Error bars represent s.d. values from three independent experiments. ( c ) Cellular extracts from synchronized Control HeLa and Ssu72 knockdown (Ssu72 KD) cells were immunoprecipitated with normal immunoglobulin G (IgG) or an anti-SA2 antibody and immunoprecipitates were analysed by immunoblotting with anti-phospho-serine and anti-SA2 antibodies. ( d ) Synchronized cells were separated into non-chromatin supernatant (Supt) and chromatin (Chro) fractions, resolved by SDS–PAGE, and immunoblotted with anti-SA2, anti-Erk1, anti-H3 and anti-Ssu72 antibodies. Full size image Aurora B binds to and phosphorylates Ssu72 in vitro The amino-acid sequence of Ssu72 included potential phosphorylation sites for the Aurora B kinase and a polo-box binding motif recognized by Plk1 (ref. 31 ). This raises the possibility that Aurora B and/or Plk1 kinase could phosphorylate Ssu72, thereby contributing to its activity and function. For the determination of the potential interaction between Ssu72 and the Aurora B and/or Plk1 kinase, HeLa cells were synchronized by double-thymidine treatment and released into the G2 phase or cultured in the presence of nocodazole, which promotes mitosis-specific phosphorylation. Cell extracts were immunoprecipitated with an anti-Ssu72 antibody and analysed by immunoblotting. Interestingly, higher levels of Aurora B were present in the complex formed with Ssu72, particularly in nocodazole-treated cells, whereas Plk1 was weakly associated with Ssu72 ( Fig. 3a ). Subsequent analyses revealed that Aurora B proteins formed a complex with endogenous Ssu72, as well as with inner centromere protein (INCENP), which is a regulatory protein of the chromosome passenger complex and involved in the regulation of Aurora B kinase ( Fig. 3b ). In addition, according to in vitro binding assays, Ssu72 interacted with Aurora B, and in particular, Aurora B was bound to the central (amino acids 61–194) and COOH-terminal (amino acids 121–194) domains of Ssu72 ( Fig. 3c,d ). These results indicate that Ssu72 forms a complex with Aurora B kinase in vitro and in vivo . 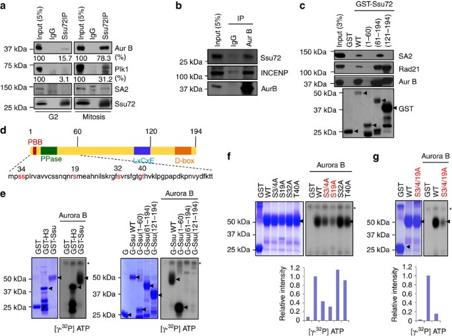Figure 3: Aurora B binds to and phosphorylates Ssu72in vitro. (a) Cellular extracts from synchronized HeLa cells were immunoprecipitated with normal immunoglobulin G (IgG) or an anti-Ssu72 antibody, and immunoprecipitates were analysed by immunoblotting with antibodies indicated. The binding intensity of co-immunoprecipitated protein relative to the input control protein was quantified by ImageJ software (http://www.rsb.info.nih.gov/ij). (b) HeLa cell extracts were immunoprecipitated with normal IgG or Aurora B antibody, and immunoprecipitates were analysed by immunoblotting with anti-Ssu72, anti-INCENP and anti-Aurora B antibodies. (c) HeLa cell extracts were incubated with beads bound to the GST alone or a series of GST-fused Ssu72 deletion mutants (amino acids 1–60, 61–120 and 121–194). Bound proteins were resolved and immunoblotted with anti-SA2, anti-Rad21, anti-Aurora B and anti-GST antibodies. The arrows denote purified GST and GST-fused Ssu72 proteins, respectively. (d) Schematic representation of human Ssu72 functional domains and putative phosphorylation sites in the N-terminal domain. (e) Purified GST, GST-Histone 3 (H3, positive control) or GST-Ssu72 WT proteins were incubated with the recombinant Aurora B kinase in the presence of [γ32P]ATP, resolved by SDS–PAGE, and analysed by autoradiography (left panels). Similarly, purified N-terminal (1–60), middle (61–120) or C-terminal (121–194) domains of GST-Ssu72 were incubated with recombinant Aurora B (right panels). (fandg) Purified GST, GST-Ssu72 WT, GST-Ssu72 S3/4A, GST-Ssu72 S19A, GST-Ssu72 S32A, GST-Ssu72 T40A and GST-Ssu72 S3/4/19A proteins were incubated with recombinant Aurora B in the presence of [γ32P]ATP, resolved by SDS–PAGE, and analysed by autoradiography. The graphs show the relative intensities of radiolabelled GST-Ssu72 proteins. Figure 3: Aurora B binds to and phosphorylates Ssu72 in vitro . ( a ) Cellular extracts from synchronized HeLa cells were immunoprecipitated with normal immunoglobulin G (IgG) or an anti-Ssu72 antibody, and immunoprecipitates were analysed by immunoblotting with antibodies indicated. The binding intensity of co-immunoprecipitated protein relative to the input control protein was quantified by ImageJ software ( http://www.rsb.info.nih.gov/ij ). ( b ) HeLa cell extracts were immunoprecipitated with normal IgG or Aurora B antibody, and immunoprecipitates were analysed by immunoblotting with anti-Ssu72, anti-INCENP and anti-Aurora B antibodies. ( c ) HeLa cell extracts were incubated with beads bound to the GST alone or a series of GST-fused Ssu72 deletion mutants (amino acids 1–60, 61–120 and 121–194). Bound proteins were resolved and immunoblotted with anti-SA2, anti-Rad21, anti-Aurora B and anti-GST antibodies. The arrows denote purified GST and GST-fused Ssu72 proteins, respectively. ( d ) Schematic representation of human Ssu72 functional domains and putative phosphorylation sites in the N-terminal domain. ( e ) Purified GST, GST-Histone 3 (H3, positive control) or GST-Ssu72 WT proteins were incubated with the recombinant Aurora B kinase in the presence of [γ 32 P]ATP, resolved by SDS–PAGE, and analysed by autoradiography (left panels). Similarly, purified N-terminal (1–60), middle (61–120) or C-terminal (121–194) domains of GST-Ssu72 were incubated with recombinant Aurora B (right panels). ( f and g ) Purified GST, GST-Ssu72 WT, GST-Ssu72 S3/4A, GST-Ssu72 S19A, GST-Ssu72 S32A, GST-Ssu72 T40A and GST-Ssu72 S3/4/19A proteins were incubated with recombinant Aurora B in the presence of [γ 32 P]ATP, resolved by SDS–PAGE, and analysed by autoradiography. The graphs show the relative intensities of radiolabelled GST-Ssu72 proteins. Full size image To determine whether the Aurora B kinase could phosphorylate Ssu72, the purified glutathione S -transferase (GST) or GST-Ssu72 and histone H3 were incubated with [γ 32 P] ATP and the recombinant Aurora B kinase ( Fig. 3e ). Ssu72 was clearly phosphorylated in the presence of Aurora B ( Fig. 3e ). In particular, the NH 2 -terminal domain (amino acids 1–60) containing the conserved protein phosphatase domain was efficiently phosphorylated by Aurora B. The amino-acid sequences of the Ssu72 NH 2 -terminal domain included several potential sites phosphorylated by Aurora B. For an analysis of their functionality, plasmids encoding GST-fused Ssu72 mutants were generated. Here, each of the five putative phosphorylation sites was mutated ( Fig. 3f ). For these, replacing S3/S4 or S19 with alanine (A) significantly reduced phosphorylation by Aurora B. In addition, the mutation of all three putative phosphorylation sites (S3/S4/S19A) strongly inhibited the phosphorylation of Ssu72 ( Fig. 3g ). Aurora B is associated with INCENP throughout the cell cycle and the kinase activity of Aurora B is altered by binding to the carboxy‐terminal IN box of INCENP [32] , [33] . Therefore, we examined whether INCENP affects the phosphorylation of Ssu72 by Aurora B kinase ( Supplementary Fig. S2 ). However, Aurora B efficiently phosphorylated Ssu72 in the absence of purified INCENP protein. Collectively, these results imply that Aurora B promoted Ssu72 phosphorylation and that at least three residues of Ssu72 were involved in this modification. In vivo phosphorylation of Ssu72 at Ser 19 by Aurora B Aurora B is upregulated at the protein level during mitosis and is known to have essential functions in chromosome congression to the spindle equator, chromosome segregation and cytokinesis [32] , [34] , [35] . According to this study’s initial experiments, the interaction between Aurora B and Ssu72 was markedly stronger in cells synchronized in mitosis. Here, a complementary approach was taken to analyse the mitotic phosphorylation status of Ssu72 through the use of lysates of HeLa cells stably expressing tandem affinity purification (TAP)-tagged Ssu72 that was synchronized in early mitosis. Liquid chromatography-mass spectrometry using an eluted TAP-tagged Ssu72 complex revealed several residues of the Ssu72 NH 2 -terminal domain as potential phosphorylation sites ( Supplementary Fig. S3a ). However, only the Ser 19 residue was reproducibly identified in mitotic cells that were enriched by a treatment with a microtubule inhibitor. Interestingly, this residue was strongly conserved among the different species ( Supplementary Figs. S3b, S4 ), implying the evolutionary conservation of the phosphorylation of Ssu72 at Ser 19. For the examination of whether the phosphorylation of Ssu72 at Ser 19 would be mediated by the Aurora B kinase in vivo , we raised a phospho-antibody on Ssu72 Ser 19 (pS19-Ssu72). Immunoblotting analyses revealed that the affinity-purified antibody efficiently recognized the phosphorylation of Ssu72 protein ( Supplementary Fig. S3 ). Specifically, the shRNA-mediated depletion of Ssu72 in HeLa cells reduced the level of phosphorylated Ssu72 at Ser 19 ( Fig. 4a ). Interestingly, although the pS19‐Ssu72 antibodies specifically recognized GST‐Ssu72 WT, they did not recognize GST-Ssu72 mutants (Ssu72 S19A, S19G and S19E), that were incubated with purified Aurora B ( Supplementary Fig. S3c ). However, this antibody failed to recognize the proteins in the S-phase and the mitotic HeLa extracts that were incubated with the lambda protein phosphatase ( Supplementary Fig. S3d ). Importantly, the phosphorylation of Ssu72 was markedly increased in mitotic extracts compared with the S and G2 phase HeLa extracts ( Supplementary Fig. S3e ). The phosphorylated levels of Ssu72 were very low at the G1/S boundary but gradually increased in late S or G2, peaked in late mitosis (11 h after release) and then sharply decreased in the next G1 phase ( Fig. 4b ). Furthermore, synchronized HeLa cells either treated with ZM447439, an Aurora B kinase selective inhibitor or transfected with Aurora B RNAi (siAur B 3′untranslated region) failed to be recognized by the pS19-Ssu72 antibodies ( Fig. 4c,d and Supplementary Fig. S3f ). However, the overexpression of HA‐tagged Aurora B in the endogenous Aurora B‐depleted HeLa cells significantly recovered the phosphorylation of Ssu72 at the Ser 19 residue. Together, these results indicate that the phosphorylation of Ssu72 at Ser 19 was specifically mediated by the Aurora B kinase during G2 and mitosis. 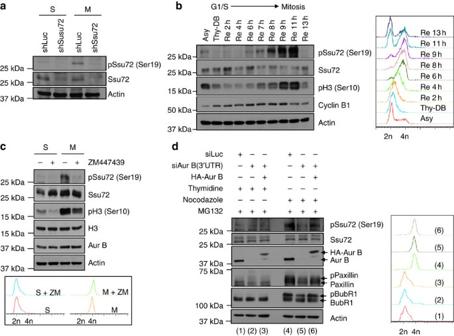Figure 4: Phosphorylation of Ssu72 by Aurora B kinasein vivo. (a) HeLa cells were transfected with shLuc or shSsu72. At 12 h post transfection, cells were synchronized in S-phase by hydroxyl urea or mitosis by nocodazole treatment and immunoblotted with indicated antibodies. (b) HeLa cells were synchronized at the G1-S boundary by Thy-DB, and then released with fresh media. At the indicated times, cells were harvested and immunoblotted with anti-Ssu72 phospho-serine 19 (pSsu72), anti-Ssu72, anti-phospho-H3 serine 10 (pH3), anti-Cyclin B1 and anti-Actin antibodies (left). Asynchronized and synchronized cells were stained with propidium iodide and analysed by flow cytometry (right). (c) Synchronised HeLa cells were further incubated in the absence or presence of 4 μM ZM447439 (Aurora B kinase inhibitor) for 2 h and immunoblotted with antibodies indicated. Synchronized cells were analysed by flow cytometry. (d) HeLa cells were transfected with indicated plasmids, and at 24 h post transfection, cells were synchronized in the S-phase or mitosis and treated with MG132. Cells were harvested and immunoblotted with antibodies as indicated (left). Transfected cells were analysed by flow cytometry (right). Figure 4: Phosphorylation of Ssu72 by Aurora B kinase in vivo . ( a ) HeLa cells were transfected with shLuc or shSsu72. At 12 h post transfection, cells were synchronized in S-phase by hydroxyl urea or mitosis by nocodazole treatment and immunoblotted with indicated antibodies. ( b ) HeLa cells were synchronized at the G1-S boundary by Thy-DB, and then released with fresh media. At the indicated times, cells were harvested and immunoblotted with anti-Ssu72 phospho-serine 19 (pSsu72), anti-Ssu72, anti-phospho-H3 serine 10 (pH3), anti-Cyclin B1 and anti-Actin antibodies (left). Asynchronized and synchronized cells were stained with propidium iodide and analysed by flow cytometry (right). ( c ) Synchronised HeLa cells were further incubated in the absence or presence of 4 μM ZM447439 (Aurora B kinase inhibitor) for 2 h and immunoblotted with antibodies indicated. Synchronized cells were analysed by flow cytometry. ( d ) HeLa cells were transfected with indicated plasmids, and at 24 h post transfection, cells were synchronized in the S-phase or mitosis and treated with MG132. Cells were harvested and immunoblotted with antibodies as indicated (left). Transfected cells were analysed by flow cytometry (right). Full size image Ser 19 phosphorylation inhibits Ssu72 phosphatase activity To determine whether the phosphorylation of Ssu72 by Aurora B would influence its phosphatase activity, GST-Ssu72 WT was incubated with the recombinant Aurora B kinase in the presence of cold ATP. The phosphatase activity of phosphorylated GST-Ssu72 was measured by monitoring the production of p -nitrophenylate from p -nitrophenyl phosphate. Interestingly, the phosphatase activity of GST-Ssu72 was significantly reduced following phosphorylation by Aurora B ( Fig. 5a ), indicating that the phosphorylation of Ssu72 by the Aurora B kinase downregulated its phosphatase activity. To further examine the effect of Ssu72 phosphorylation, particularly at Ser 19 on its phosphatase activity, phosphomimetic mutants of GST-Ssu72 were constructed by replacing S3/S4 and/or S19 with glutamate (E) as indicated and were analysed to measure the phosphatase activity of a series of GST-Ssu72 WT and mutants ( Fig. 5b ). Importantly, in vitro phosphatase assays revealed that a phosphomimetic Ssu72 mutant (Ssu72 S19E) almost completely abolished phosphatase activity as much as a phosphatase-dead mutant of Ssu72 (C12S), whereas the mutations of Ser 3 and Ser 4 with Glu (Ssu72 S3/4E) retained phosphatase activity ( Fig. 5b ). 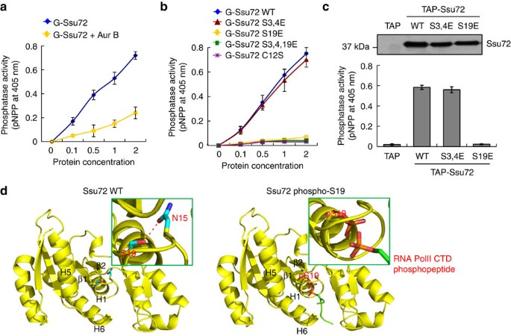Figure 5: Aurora B inhibits the phosphatase activity of Ssu72 through phosphorylation at Ser 19. (a) Purified GST-Ssu72 was reacted with the recombinant Aurora B kinase in the presence of cold ATP. GST-Ssu72 WT phosphorylatedin vitrowas incubated in a phosphatase buffer containing para-nitrophenyl phosphate (pNPP). The reaction was stopped by the addition of NaOH solution, and phosphatase activity was measured at 405 nm using an enzyme-linked immunosorbent assay reader. Error bars indicate s.d. from three independent experiments. (b) Purified GST-fused Ssu72 WT, Ssu72 phosphomimetic mutants (GST-Ssu72 S3/4E, GST-Ssu72 S19E and GST-Ssu72 S3/4/19E), Ssu72 phosphatase-inactive mutants (GST-Ssu72 C12S, negative control) were reacted with pNPP solution. Error bars display s.d. from three independent experiments. (c) HeLa cells transfected with expression plasmids encoding the TAP epitope, TAP-Ssu72 WT, TAP-Ssu72 S3/4E, TAP-Ssu72 S19E. At 48 h after transfection, cells were harvested and purified using agarose beads bound to protein S. Equal amounts of purified TAP-tagged proteins were reacted with pNPP solution. Error bars indicate s.d. from three independent experiments. (d) Structural modelling of human Ssu72 WT (left) and Ssu72 phospho-S19 (right). Enlarged panel shows the hydrogen bonding between S19 and N15 (left). Right panel shows conformational hindrance between pS19 and RNAPII CTD Ser 5 phosphopeptide (pS5). Figure 5: Aurora B inhibits the phosphatase activity of Ssu72 through phosphorylation at Ser 19. ( a ) Purified GST-Ssu72 was reacted with the recombinant Aurora B kinase in the presence of cold ATP. GST-Ssu72 WT phosphorylated in vitro was incubated in a phosphatase buffer containing para-nitrophenyl phosphate (pNPP). The reaction was stopped by the addition of NaOH solution, and phosphatase activity was measured at 405 nm using an enzyme-linked immunosorbent assay reader. Error bars indicate s.d. from three independent experiments. ( b ) Purified GST-fused Ssu72 WT, Ssu72 phosphomimetic mutants (GST-Ssu72 S3/4E, GST-Ssu72 S19E and GST-Ssu72 S3/4/19E), Ssu72 phosphatase-inactive mutants (GST-Ssu72 C12S, negative control) were reacted with pNPP solution. Error bars display s.d. from three independent experiments. ( c ) HeLa cells transfected with expression plasmids encoding the TAP epitope, TAP-Ssu72 WT, TAP-Ssu72 S3/4E, TAP-Ssu72 S19E. At 48 h after transfection, cells were harvested and purified using agarose beads bound to protein S. Equal amounts of purified TAP-tagged proteins were reacted with pNPP solution. Error bars indicate s.d. from three independent experiments. ( d ) Structural modelling of human Ssu72 WT (left) and Ssu72 phospho-S19 (right). Enlarged panel shows the hydrogen bonding between S19 and N15 (left). Right panel shows conformational hindrance between pS19 and RNAPII CTD Ser 5 phosphopeptide (pS5). Full size image For a comparison of phosphatase activity between the wild-type and phosphomimetic mutant of Ssu72 in vivo , phosphatase activity was measured using equal amounts of purified Ssu72 WT and mutants from HeLa cells transfected with an expression plasmid encoding TAP-tagged Ssu72 WT, S3/4E, or S19E ( Fig. 5c ). As expected, the phosphatase activity of Ssu72 S19E dramatically and almost completely inhibited phosphatase activity in vivo (although this was not the case for Ssu72 S3/4E), indicating that the phosphorylation of Ssu72 Ser 19 by the Aurora B kinase downregulated its phosphatase activity. A recent phosphoproteomic analysis using multidimensional liquid chromatography-mass spectrometry identified that the phosphorylation of hsSsu72 on Ser 3 and Ser 4 is abundant in undifferentiated human embryonic stem cells [36] . This suggests that the hypophosphoryation of hsSsu72 may alter its biochemical property and function, thereby facilitating cell division and differentiation. However, this study’s results indicate that the mutations of Ssu72 Ser 3 and Ser 4 influenced neither the phosphatase activity of Ssu72 nor the sister chromatid arm cohesion. It is important to note that a residue Ser 19 is located close to helix 1 and is also surrounded by two parallel β‐sheets (β1–2) in the human Ssu72 protein structure [37] . The residue Ser 19 seems to contribute to the stabilization of the Ssu72 structure by hydrogen bonding with Asn 15 (N15) ( Fig. 5d , left). To confirm the correlation between the phosphorylation at Ser 19 and the phosphatase activity of Ssu72, we remodelled the crystal structure of Ssu72 protein based on the Ssu72‐RNAPII CTD complex structure (PDB ID 3O2Q) [37] . As shown in Fig. 5d , the structural analysis shows that the phosphate group of a phospho‐Ser 19 (pS19) is sufficiently close to a RNAPII CTD Ser 5 phosphopeptide to cause steric hindrance and charge repulsion, indicating that it is energetically unfavourable for the CTD phosphopeptide to bind to the Ssu72. Thus, the phosphorylation of Ssu72 at Ser 19 may influence the protein configuration and the phosphatase activity of Ssu72. We then generated the non-phosphorylatable mutant of Ssu72 (S19A) and examined its phosphatase activity through in vitro and in vivo phosphatase assay. Unexpectedly, we found that the phosphatase activity of the Ssu72 phospho‐dead mutant (S19A) decreased by ~10-fold compared with that of Ssu72 WT ( Fig. 6a,b ). This is in sharp contrast to the expected phosphatase activity of the Ssu72 non-phosphorylatable mutant. Based on our structural analysis, although the mutation of Ser 19 to Ala would not cause steric hindrance and charge repulsion between a Ssu72 pS19 and the CTD pS5, allowing the binding of RNAPII CTD phosphopeptide to the Ssu72, this mutation appears to cause the elimination of hydrogen bonding between the Ser 19 and the Asn 15 (N15). This therefore generates an empty space in the inner region, which contributes to the destabilization of the Ssu72 non-phosphorylatable mutant ( Fig. 6c , middle panel). Furthermore, the hydrophobic side chain of the Ala residue interferes with the access of RNAPII CTD phosphopeptide to the phosphatase active site of Ssu72. To avoid the influence of the hydrophobic side chain, we therefore generated a new non-phosphorylatable mutant of Ssu72 by substituting Ser 19 for Gly (S19G), which does not have the hydrophobic side chain ( Fig. 6c , right panel). Interestingly, although the phosphatase activity of the Ssu72 S19G mutant was significantly enhanced, it was not as enhanced as that of Ssu72 WT ( Fig. 6a,b ). This indicates that the mutation of Ssu72 at Ser 19 is highly inclined to cause the conformational change and to downregulate the phosphatase activity of Ssu72. However, the Ssu72 S19G mutant significantly retained the phosphatase activity approximately threefold greater than the Ssu72 S19A mutant possibly due to the absence of a hydrophobic side chain. In the case of a phosphomimetic Ssu72 S19E mutant, the mutation of Ser 19 to Glu (E19) causes a steric hindrance and charge repulsion between the side chain of E19 and the phosphate group of RNAPII CTD pS5 ( Fig. 6c , left panel). This conformational change strongly underlines our earlier results of the phosphates’ assay showing that the Ssu72 S19E mutant completely abolished its phosphatase activity. 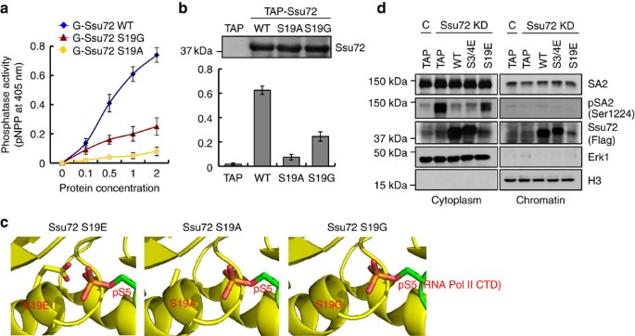Figure 6: Characterization of Ssu72 phosphorylation at Ser 19. (a) Purified GST-Ssu72 WT and non-phosphorylatable mutants (GST-Ssu72 S19A and GST-Ssu72 S19G) were reacted with pNPP solution. Error bars indicate s.d. from five independent experiments. (b) HeLa cells transfected with TAP, TAP-Ssu72 WT, TAP-Ssu72 S19A and TAP-Ssu72 S19G plasmids. At 48 h after transfection, cells were harvested and purified using protein S agarose beads. Equal amounts of purified TAP-tagged proteins were reacted with pNPP solution. Error bars indicate s.d. from three independent experiments. (c) Schematic drawing of the structure of human Ssu72 S19E, S19A and S19G mutants. These models illustrate the conformational difference between the phosphomimetic mutant (S19E) and the non-phosphorylatable mutants (S19A and S19G) of Ssu72 in the configuration with the RNAPII CTD Ser 5 phosphopeptide. (d) Control HeLa cells (C) or Ssu72 knockdown HeLa cells (Ssu72 KD) were transfected with a TAP, TAP-Ssu72 WT, TAP-Ssu72 S3/4E or TAP-Ssu72 S19E expression plasmid. Transfected cells were synchronized in mitosis by the Thy-DB and the release into fresh media and then incubated in the presence of nocodazole for 4 h. Cellular extracts were separated into soluble non-chromatin cytoplasmic and insoluble chromatin fractions and immunoblotted with anti-SA2, anti-pSA2 (Ser 1224), anti-Flag, anti-Erk1 and anti-Histone 3 antibodies. Figure 6: Characterization of Ssu72 phosphorylation at Ser 19. ( a ) Purified GST-Ssu72 WT and non-phosphorylatable mutants (GST-Ssu72 S19A and GST-Ssu72 S19G) were reacted with pNPP solution. Error bars indicate s.d. from five independent experiments. ( b ) HeLa cells transfected with TAP, TAP-Ssu72 WT, TAP-Ssu72 S19A and TAP-Ssu72 S19G plasmids. At 48 h after transfection, cells were harvested and purified using protein S agarose beads. Equal amounts of purified TAP-tagged proteins were reacted with pNPP solution. Error bars indicate s.d. from three independent experiments. ( c ) Schematic drawing of the structure of human Ssu72 S19E, S19A and S19G mutants. These models illustrate the conformational difference between the phosphomimetic mutant (S19E) and the non-phosphorylatable mutants (S19A and S19G) of Ssu72 in the configuration with the RNAPII CTD Ser 5 phosphopeptide. ( d ) Control HeLa cells (C) or Ssu72 knockdown HeLa cells (Ssu72 KD) were transfected with a TAP, TAP-Ssu72 WT, TAP-Ssu72 S3/4E or TAP-Ssu72 S19E expression plasmid. Transfected cells were synchronized in mitosis by the Thy-DB and the release into fresh media and then incubated in the presence of nocodazole for 4 h. Cellular extracts were separated into soluble non-chromatin cytoplasmic and insoluble chromatin fractions and immunoblotted with anti-SA2, anti-pSA2 (Ser 1224), anti-Flag, anti-Erk1 and anti-Histone 3 antibodies. Full size image To further examine the hyperphosphorylation or dephosphorylation of SA2 by overexpressing the Ssu72 WT, S3/4E or S19E mutant in the Ssu72-depleted cells, the shRNA-insensitive version of TAP-tagged Ssu72 WT, S3/4E or S19E mutant was transfected into the Ssu72-depleted HeLa cells, and the cells were synchronized in mitosis. Extracts from these synchronized HeLa cells were separated into chromatin and non-chromatin cytoplasmic fractions, and these fractions were immunoblotted with anti-SA2, anti-phospho SA2 S1224 (which recognizes SA2 phosphorylated at Ser 1224) and anti-Flag antibodies ( Fig. 6d ). As expected, the level of the hyperphosphorylated form of SA2 in the non-chromatin cytoplasmic fractions decreased sharply in cells transfected with Ssu72 WT or S3/4E, whereas it was significantly retained in cells overexpressing Ssu72 S19E. The results of a comparison of the expression level or stability of Ssu72 S19E with that of Ssu72 WT or S3/4E indicate that the level of hyperphosphorylated SA2 in Ssu72 S19E-overexpressing cells was retained almost as much as that in the TAP-transfected cells. Together, these results indicate that the phosphorylation of Ssu72 by Aurora B kinase downregulated its phosphatase activity. Ssu72 phosphorylation is essential for cohesin dissociation For an examination of the effect of Aurora B-mediated Ssu72 phosphorylation on sister chromatid arm cohesion, HeLa cells were transfected with luciferase shRNA (control), Aurora B shRNA or Ssu72 shRNA and treated with colcemid. Sister chromatid cohesion was analysed by chromosome spreading ( Fig. 7a–c ). Four types of mitotic chromosome patterns were observed: ‘open’ (complete loss of arm cohesion), ‘partially open’ (partial loss of arm cohesion), ‘closed’ (cohesed arms) and ‘condensed (closed)’ (condensed chromosomes and cohesed arms). As shown in Fig. 7c , the shLuciferase (shLuc)-transfected control cells treated with a microtubule inhibitor showed mixed-type mitotic chromosome spreads composed of open (about 50%), partially open (40%) and closed (10%) conformations. For the condition in which the depletion of Ssu72 increased the population of completely open arms, it also reduced partially open and closed arms. On the other hand, the depletion of Aurora B dramatically increased closed arms (including condensed arms), and sharply reduced open and partially open arms ( Fig. 7c ). Interestingly, the double depletion of Ssu72 and Aurora B significantly reduced the closed type, but the open and partially open phenotypes remarkably increased ( Fig. 7c ). Consistently, further biochemical analyses using fractionated cellular extracts revealed that the depletion of Aurora B in control cells led to the significant increase of Rad21 and SA2 levels in the chromatin fractions of control cells ( Supplementary Fig. S5 ). However, the depletion of Aurora B failed to rescue the dissociation of Rad21 and SA2 proteins from the chromatin of Ssu72-depleted cells. Next, we generated HeLa cells stably expressing shAurora B (Aurora B depletion) and HA-tagged Aurora B (Aurora B overexpression) and then depleted Ssu72 by shRNA transfection ( Supplementary Fig. S6 ). As expected, the inhibition of Ssu72 expression in the Aurora B-depleted cells showed a marked increase of open phenotype, whereas the depletion of Ssu72 in Aurora B-overexpressed cells did not show a significant change in the chromosome arm cohesion phenotypes compared with the control cells. Collectively, the notion that Ssu72-mediated maintenance of chromosome arm cohesion is overridden by Aurora B expression indicates that Aurora B, as an upstream regulator, targets Ssu72 to regulate the dissociation of arm cohesion. 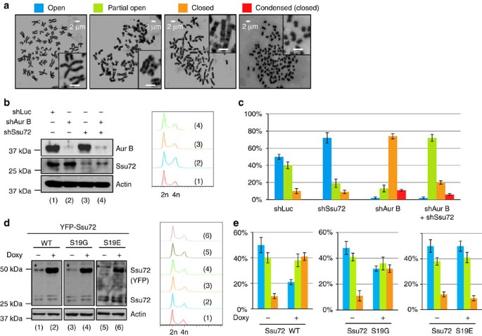Figure 7: Phosphorylation of Ssu72 by Aurora B is essential for the dissociation of chromosome arm cohesion. (a–c) HeLa cells were cotransfected with shLuc, shSsu72 and shAur B, either singly or in combination. At 44 h after transfection, the cells were treated with 0.04 mg ml−1colcemid and cultured for another 4 h. (a) Mitotic chromosomes were spread and visualised by Giemsa staining. Scale bars represent 2 μm. (b) Subsequently, cell extracts were immunoblotted with anti-Aurora B, anti-Ssu72 and anti-Actin antibodies. (c) More than 600 mitotic cells were randomly examined and categorised based on the resolution pattern of sister chromatid cohesion, as shown ina. All data were calculated from three independent experiments (mean±s.d.). (dande) Inducible HeLa cells expressing YFP-Ssu72 WT, YFP-Ssu72 S19G or YFP-Ssu72 S19E were cultured in the absence (−) or presence (+) of 2 μg ml−1doxycycline (Doxy) and further treated with colcemid. (d) Cellular extracts were immunoblotted with anti-YFP, anti-Ssu72 and anti-Actin antibodies. (e) The percentage of mitotic chromosome spreading was calculated from at least 400 cells per transfectant and from three independent experiments (mean±s.d.). Figure 7: Phosphorylation of Ssu72 by Aurora B is essential for the dissociation of chromosome arm cohesion. ( a – c ) HeLa cells were cotransfected with shLuc, shSsu72 and shAur B, either singly or in combination. At 44 h after transfection, the cells were treated with 0.04 mg ml −1 colcemid and cultured for another 4 h. ( a ) Mitotic chromosomes were spread and visualised by Giemsa staining. Scale bars represent 2 μm. ( b ) Subsequently, cell extracts were immunoblotted with anti-Aurora B, anti-Ssu72 and anti-Actin antibodies. ( c ) More than 600 mitotic cells were randomly examined and categorised based on the resolution pattern of sister chromatid cohesion, as shown in a . All data were calculated from three independent experiments (mean±s.d.). ( d and e ) Inducible HeLa cells expressing YFP-Ssu72 WT, YFP-Ssu72 S19G or YFP-Ssu72 S19E were cultured in the absence (−) or presence (+) of 2 μg ml −1 doxycycline (Doxy) and further treated with colcemid. ( d ) Cellular extracts were immunoblotted with anti-YFP, anti-Ssu72 and anti-Actin antibodies. ( e ) The percentage of mitotic chromosome spreading was calculated from at least 400 cells per transfectant and from three independent experiments (mean±s.d.). Full size image Doxycycline-inducible HeLa cells stably expressing YFP-tagged Ssu72 WT, S19G or S19E were generated and treated with colcemid ( Fig. 7d,e , and Supplementary Fig. S6c–f ). In contrast to the behaviour of Ssu72-depleting cells described earlier, doxycycline-induced cells expressing Ssu72 WT showed a marked increase in closed phenotypes compared with the uninduced control cells. Interestingly, cells expressing Ssu72 S19G mutant showed a moderate increase in closed phenotypes compared with the uninduced cells ( Fig. 7e ), which is consistent with earlier evidence obtained from structural analysis and phosphatase assay. However, cells expressing Ssu72 S19E mutant failed to increase the population of the closed phenotype and showed chromosome conformations very similar to those for the uninduced control or Ssu72 WT cells ( Fig. 7e ), indicating that expression of the Ssu72 S19G non-phosphorylatable mutant but not of the phosphomimetic S19E mutant is able to overcome the dissociation of sister chromatid arm cohesion in Ssu72-depleted cells. Furthermore, the overexpression of the Ssu72 WT or S19G mutant in cells that were depleting both Aurora B and Ssu72 expressions significantly recovered the resolution of arm cohesion, whereas the overexpression of Ssu72 S19E mutant did not ( Supplementary Fig. S6f ). Collectively, these results suggest that the Aurora B-mediated Ser 19 phosphorylation of Ssu72 is an important process in regulating sister chromatid arm cohesion. Ssu72 phosphorylation enhances its degradation In the initial attempt to examine the subcellular colocalization of Ssu72 and Aurora B in mitotic cells, HeLa cells were transfected with an expression plasmid encoding Myc epitope-tagged Aurora B and immunostained ( Fig. 8a ). Unexpectedly, the colocalization of Ssu72 and Aurora B were difficult to detect because cells overexpressing Aurora B showed the dramatic destabilization of Ssu72. Similarly, an immunoblotting analysis revealed that the overexpression of Aurora B sharply reduced the stability of Ssu72 ( Fig. 8b ). We then transfected the HeLa cells with control shLuc or shAurora B and immunostained them. In contrast to the phenotypes of cells overexpressing Aurora B, the depletion of Aurora B significantly increased the protein level of endogenous Ssu72, particularly in the mitotic phase of cells ( Fig. 8c ). In addition, although the protein level of the Ssu72 phosphomimetic mutant (Ssu72 S19E) was highly unstable, it was markedly recovered by a treatment with MG132, a proteosome inhibitor. In contrast, the protein level of Ssu72 WT was highly stable and almost constant throughout the treatment ( Fig. 8d ), indicating that the phosphorylation of Ssu72 by Aurora B destabilized its protein stability. 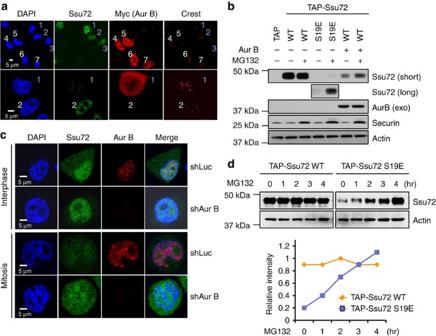Figure 8: The phosphorylation of Ssu72 by Aurora B reduces its stability. (a) HeLa cells were transfected with the Myc-Aurora B plasmid and stained with anti-Ssu72 (green) and anti-Myc (red) antibodies and anti-CREST serum (purple). The numbers indicate different cells in the same cover glass. Scale bars represent 5 μm. (b) HeLa cells were cotansfected with TAP, TAP-Ssu72 WT or TAP-Ssu72 S19E and Myc-Aurora B expression plasmids in combination. At 40 h after transfection, the cells were further cultured in the absence or presence of MG132 for 6 h, and cellular extracts were immunoblotted with indicated antibodies. (c) HeLa cells were transfected with the shLuc or shAur B and stained with anti-Ssu72 (green) and anti-Aurora B (red) antibodies. Scale bars represent 5 μm. (d) HeLa cells were transfected with expression plasmids encoding TAP-Ssu72 WT or TAP-Ssu72 S19E and treated with MG132 for indicated times. Cellular extracts were immunoblotted with anti-Ssu72 and anti-Actin antibodies. The graph shows the relative intensities of TAP-Ssu72 WT and TAP-Ssu72 S19E based on densitometric scanning analyses. Figure 8: The phosphorylation of Ssu72 by Aurora B reduces its stability. ( a ) HeLa cells were transfected with the Myc-Aurora B plasmid and stained with anti-Ssu72 (green) and anti-Myc (red) antibodies and anti-CREST serum (purple). The numbers indicate different cells in the same cover glass. Scale bars represent 5 μm. ( b ) HeLa cells were cotansfected with TAP, TAP-Ssu72 WT or TAP-Ssu72 S19E and Myc-Aurora B expression plasmids in combination. At 40 h after transfection, the cells were further cultured in the absence or presence of MG132 for 6 h, and cellular extracts were immunoblotted with indicated antibodies. ( c ) HeLa cells were transfected with the shLuc or shAur B and stained with anti-Ssu72 (green) and anti-Aurora B (red) antibodies. Scale bars represent 5 μm. ( d ) HeLa cells were transfected with expression plasmids encoding TAP-Ssu72 WT or TAP-Ssu72 S19E and treated with MG132 for indicated times. Cellular extracts were immunoblotted with anti-Ssu72 and anti-Actin antibodies. The graph shows the relative intensities of TAP-Ssu72 WT and TAP-Ssu72 S19E based on densitometric scanning analyses. Full size image To verify whether the reduced stability of Ssu72 by the Aurora B-mediated phosphorylation was due to ubiquitin-dependent degradation, a series of in vivo ubiquitination assays was performed. First, HeLa cells were transfected with a TAP-Ssu72 WT and/or Aurora B expression plasmid individually or in combination with HA-Ubiquitin and cultured in the presence of nocodazole ( Fig. 9a ). Immunoblotting analyses using a purified TAP-Ssu72 complex demonstrated that the overexpression of Aurora B severely polyubiquitinated Ssu72 ( Fig. 9a,b ). However, the polyubiquitination of Ssu72 was not detectable in the control cells and kinase-dead Aurora B mutant-overexpressing cells ( Fig. 9a,b ). Second, we compared the degree of ubiquitinational degradation between the Ssu72 WT and the Ssu72 mutants. Although the mutation of Ser 19 seems to be highly susceptible to the conformational change and to reduce the protein stability, the non-phosphorylatable mutants (Ssu72 S19A and Ssu72 S19G) were markedly less polyubiquitinated than the phosphomimetic mutant (Ssu72 S19E). On the other hand, Ssu72 WT was clearly evident and showed no significant polyubiquitination, indicating that the phosphorylation of Ssu72 by Aurora B triggered ubiquitin-dependent degradation ( Fig. 9c ). Taken together, these results suggest that the Aurora B-mediated phosphorylation of Ssu72 is an important molecular process in regulating sister chromatid arm cohesion during early mitosis. 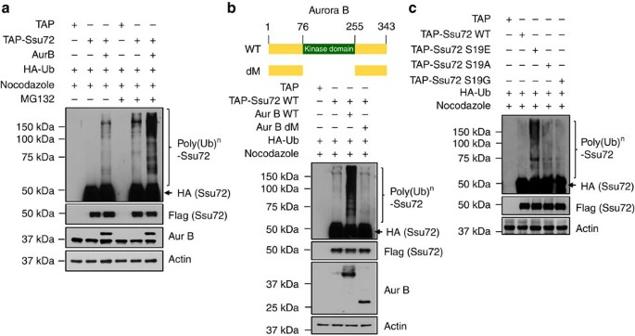Figure 9: The phosphorylation of Ssu72 by Aurora B triggers ubiquitin-dependent degradation. (a–c) HeLa cells were transfected with indicated plasmids and harvested for anin vivoubiquitination assay. (a) HeLa cells were cotansfected with TAP or TAP-Ssu72 WT or Myc-Aurora B and HA-ubiquitin expression plasmids in combination. At 24 h after transfection, cells were cultured in the presence of 330 nM nocodazole for 16 h. MG132 (25 mM) was added to mitotic cells after the 12-h incubation in nocodazole. Cellular extracts were immunblotted with anti-HA, anti-Flag, anti-Aurora B and anti-Actin antibodies. Transfected cells were analysed by flow cytometry. (b) Schematic diagram of the Aurora B WT and kinase domain deletion mutant (dM). HeLa cells were transfected with indicated plasmids, and at 24 h after transfection, cells were cultured in the presence of 330 nM nocodazole and 10 mM MG132 for 16 h. Harvested cellular extracts were immunblotted with antibodies indicated. (c) HeLa cells were cotransfected with TAP, TAP-Ssu72 WT or TAP-Ssu72 S19E and HA-ubiquitin expression plasmids, treated with 330 nM nocodazole for 16 h, and 25 mM MG132 was added to mitotic cells after the 12-h incubation in nocodazole. Extracts were analyzed by an immunoblotting analysis. Figure 9: The phosphorylation of Ssu72 by Aurora B triggers ubiquitin-dependent degradation. ( a – c ) HeLa cells were transfected with indicated plasmids and harvested for an in vivo ubiquitination assay. ( a ) HeLa cells were cotansfected with TAP or TAP-Ssu72 WT or Myc-Aurora B and HA-ubiquitin expression plasmids in combination. At 24 h after transfection, cells were cultured in the presence of 330 nM nocodazole for 16 h. MG132 (25 mM) was added to mitotic cells after the 12-h incubation in nocodazole. Cellular extracts were immunblotted with anti-HA, anti-Flag, anti-Aurora B and anti-Actin antibodies. Transfected cells were analysed by flow cytometry. ( b ) Schematic diagram of the Aurora B WT and kinase domain deletion mutant (dM). HeLa cells were transfected with indicated plasmids, and at 24 h after transfection, cells were cultured in the presence of 330 nM nocodazole and 10 mM MG132 for 16 h. Harvested cellular extracts were immunblotted with antibodies indicated. ( c ) HeLa cells were cotransfected with TAP, TAP-Ssu72 WT or TAP-Ssu72 S19E and HA-ubiquitin expression plasmids, treated with 330 nM nocodazole for 16 h, and 25 mM MG132 was added to mitotic cells after the 12-h incubation in nocodazole. Extracts were analyzed by an immunoblotting analysis. Full size image In this study, we showed that Ssu72 is an essential modifier in regulating sister chromatid arm cohesion, a function that is clearly regulated by Aurora B kinase activity. Notably, cohesin dissociation depends on the mitotic kinases, such as Cdk1, Aurora B and Plk1 (refs 2 , 3 , 4 ) Specifically, Rad21 and SA1/SA2 became phosphorylated during mitosis, which is dependent on Plk1, and this phosphorylation inhibited the binding of cohesin to chromatin, implying that cohesin–DNA interactions might have been directly controlled by Plk1-mediated phosphorylation [2] . Similarly, previous research has suggested that the Aurora B kinase is required for the efficient dissociation of cohesin subunits from chromosome in prophase [4] . However, Aurora B kinase failed to directly phosphorylate cohesin subunit proteins, indicating that Aurora B is required for cohesin dissociation by regulating other proteins or by the indirect pathway. In addition, the role of the Aurora B kinase in regulating cohesin dissociation has yet to be clearly addressed. The results of this study indicate that Ssu72 was a direct target of the Aurora B kinase and that the phosphorylation of Ssu72 by the Aurora B kinase influenced the physiological role of Ssu72 as a cohesin-binding phosphatase. Interestingly, the inhibition of the Ssu72 expression in Aurora B-depleted cells significantly recovered the prevention of arm cohesin dissociation that was sharply induced by Aurora B depletion, indicating that Aurora B antagonized the Ssu72 function. In addition, the prevention of cohesin dissociation caused by Wapl depletion was strongly antagonized in the Ssu72-depleted cells [31] . Furthermore, there was a significant increase in the interaction between Rad21 and Wapl in Ssu72-depleted cells (Kim and Lee, an unpublished observation). In this regard, this may be an attractive model in that the recruitment of Ssu72 to the cohesin complex antagonized the interaction between cohesin subunits and Wapl. Although SA2 phosphorylation is required for efficient cohesin dissociation, recent studies of Wapl have suggested that cohesin phosphorylation is not sufficient to remove cohesins from chromosomes [5] , [6] . If Wapl is depleted, then cohesin dissociation is reduced more dramatically than after the inactivation of Aurora B and/or Plk1 (ref. 5 ). In this regard, we do not exclude the possibility that the antagonisation of SA2 phosphorylation by Ssu72 is effective but may be partially required to remove cohesins from chromosome arms. However, we believe that hyperphosphorylations of SA2 have an important role in arm cohesin resolution, because hyperphosphorylated SA2 is found only in cytoplasm (non-chromatin fractions) of both nocodazole-arrested and unperturbed cells [8] , [31] . Therefore, this result indicates that the hyperphosphorylations of SA2 in unperturbed cells are essential for the cohesin dissociation from the chromosome arm regardless of the cohesin destabilizing activity of Wapl during early mitosis. Wapl is one of the highly phosphorylated cohesin subunits and is phosphorylated by Plk1 in mitosis [38] , which suggests that the hyperphosphorylation of Wapl has an important role in the regulatory mechanism underlying the removal of arm-bound cohesins. The notion that Plk1 is a major Wapl kinase raises the interesting possibility that two mitotic kinases, Aurora B and Plk1, have the selectivity to target two reciprocal and antagonistic regulatory substrates, Ssu72 and Wapl, respectively, for chromosome arm cohesion in early mitosis. This hypothesis posits that different phosphorylation combinations of cohesin subunits (and regulatory proteins) orchestrate the sequential regulation of sister chromatid cohesion and stepwise resolution and separation during the cell cycle procession. As for the case of Ssu72, the Sgo1-PP2A complex is known to dephosphorylate the SA2 subunit in vitro [9] , [10] , and the cohesion defect caused by Sgo1 depletion can be restored by the expression of non-phosphorylatable SA2 (ref. 11 ). Therefore, Sgo1 may protect cohesins from the prophase pathway by recruiting PP2A to centromeres. Interestingly, the inhibition of the Aurora B kinase influences Sgo1 localization by causing the redistribution of Sgo1 to chromosome arms from centromeres [5] , [39] . This raises another possibility that Sgo1 may functionally cross-talk with Ssu72 at the chromosome arms in the Aurora B-depleted cells, in a nonphosphorylation-dependent manner; this requires further research. In this study, the phosphatase activity of Ssu72 was maintained until the G2 phase; it then declined sharply in mitosis, indicating that Ssu72 was involved in maintaining sister chromatid cohesion until the G2 phase ( Figs 2b and 10 ). In addition, the phosphatase activity of Ssu72 limited the premature dissociation of arm cohesins by inhibiting SA2 hyperphosphorylation before the onset of Wapl-mediated cohesin dissociation [31] Furthermore, the cohesion between sister chromatid arms in the Ssu72-depleted cells decreased in the G2 phase cells, indicating that the premature dissociation of cohesins in Ssu72-depleted cells occurred before the G2 phase. This also implies that Ssu72 facilitated the establishment of sister chromatid cohesion during DNA replication. 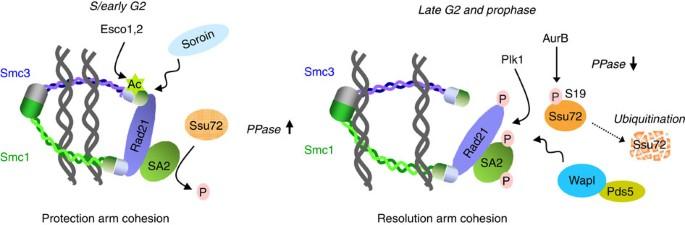Figure 10: Schematic model of the Aurora B-mediated phosphorylation of Ssu72 phosphatase in regulating sister chromatid arm cohesion. During the S and G2 phases, Ssu72 may associate with chromatin and be involved in maintaining sister chromatid arm cohesion through the process of protecting SA2 hyperphosphorylation, which may be mediated by Cdk1 and Plk1. During a similar cell cycle period, Smc3 subunits are acetylated by Esco1 and Esco2 associated with replication forks16,18. Sororin loads on chromatin depending on Smc3 acetylation and thus antagonizes the destabilization of cohesion by the Wapl–Pds5 complex22,23. Therefore, Sororin may facilitate sister chromatid cohesion by reducing the ability to inhibit Wapl–Pds5 activity. Upon the onset of mitosis, the hyperphosphorylation of Ssu72 at the Ser 19 residue by Aurora B downregulates phosphatase activity and then triggers the ubiquitinational degradation of Ssu72. As a result of this posttranslational modification of Ssu72, SA2 becomes eligible for hyperphosphorylation by Plk1, thereby inducing the dissociation of chromosome arm cohesin. Figure 10: Schematic model of the Aurora B-mediated phosphorylation of Ssu72 phosphatase in regulating sister chromatid arm cohesion. During the S and G2 phases, Ssu72 may associate with chromatin and be involved in maintaining sister chromatid arm cohesion through the process of protecting SA2 hyperphosphorylation, which may be mediated by Cdk1 and Plk1. During a similar cell cycle period, Smc3 subunits are acetylated by Esco1 and Esco2 associated with replication forks [16] , [18] . Sororin loads on chromatin depending on Smc3 acetylation and thus antagonizes the destabilization of cohesion by the Wapl–Pds5 complex [22] , [23] . Therefore, Sororin may facilitate sister chromatid cohesion by reducing the ability to inhibit Wapl–Pds5 activity. Upon the onset of mitosis, the hyperphosphorylation of Ssu72 at the Ser 19 residue by Aurora B downregulates phosphatase activity and then triggers the ubiquitinational degradation of Ssu72. As a result of this posttranslational modification of Ssu72, SA2 becomes eligible for hyperphosphorylation by Plk1, thereby inducing the dissociation of chromosome arm cohesin. Full size image Transcription by RNAPII is coupled to messenger RNA processing and chromatin modification through the C-terminal domain (CTD) of its largest subunit [40] . The RNAPII CTD is essential for viability, and partial truncation or site-specific mutation leads to specific growth defects [41] . Interestingly, the phosphorylational regulation of the CTD at serine residues (Ser 2, Ser 5 and Ser 7) is essential for transcription initiation, messenger RNA elongation and processing [42] , [43] . Recent studies have demonstrated that Ssu72 dephosphorylates both Ser 5 and Ser 7 in the RNAPII CTD, and thus has a crucial role in controlling the CTD during the transcription cycle [44] . In this study, however, it is unlikely that the downregulation of Ssu72 phosphatase activity by Aurora B-mediated phosphorylation was coupled with the transcriptional regulation by RNAPII because the phosphorylation of Ssu72 by Aurora B appeared to be restricted in the transcriptionally inactive mitotic stage of the cell cycle. How Ssu72 discriminates its substrate proteins for dephosphorylation remains unclear. However, a number of possible Ssu72 modification states may lead to diverse functions of Ssu72 in which different combinations of modifications direct the sequential requirement of the Ssu72 phosphatase during transcription and chromosome cohesion and separation cycles. It is worth noting that, according to this study’s gel filtration assays, the majority of Ssu72 from G2-arrested cells was found in the non-cohesin pool (>80%) but that low amounts of Ssu72 were cofractionated with the cohesin pool (less than 20%) ( Supplementary Fig. S7 ). This implies that limited amounts of Ssu72 made a complex with the cohesin subunits and that a majority of the soluble population of Ssu72 was involved in other activities such as transcription and RNA processing. Interestingly, in cells synchronised in mitosis, there was very little Ssu72 in the cohesin pool (less than 4%) but a substantial amount in the non-cohesin pool ( Supplementary Fig. S7 ). This discrepancy in the amounts of cohesin-bound Ssu72 between G2 and mitosis appeared to be associated with Aurora B-mediated phosphorylation and the ubiquitin-dependent degradation of Ssu72 during mitosis ( Fig. 10 ). Following mitosis, the remaining amount of Ssu72 in the non-cohesin pool (or newly synthesized Ssu72) was dephosphorylated and recycled for another round of chromosome arm cohesion. However, future research should provide a better understanding of this intriguing level of complexity. Plasmids and shRNA construction Full-length cDNA sequences of human Ssu72 genes were amplified by PCR using templates generated by reverse transcription from HeLa cell total mRNA and using oligo-dT primers. Ssu72 mutant alleles were generated by site-directed mutagenesis. cDNAs for the Ssu72 wild-type (WT) and phosphomimetic (S3/4E, S19E and S3/4/19E) and phospho-dead (S3/4A, S19A and S3/4/19A) mutant versions of Ssu72 were subcloned into YFP, TAP or GST epitope-encoding vectors, respectively. The Myc-tagged Aurora B WT and deletion mutant were provided by Ashish Jain [45] . For the shRNA synthesis, the following gene-specific sequences were generated using the pSuper vector (Oligoengine): Ssu72 shRNA, 5′-AAGACCTGTTTGATCTGATCC-3′; Aurora B shRNA, 5′-CGCGGCACTTCACAATTGATG-3′; Rad21 shRNA, 5′-GGTGAAAATGGCATTACGG-3′; and Luciferase shRNA, 5′-CTACGCGGAATACTTCGATG-3′; the 3′ untranslated region (untranslated region) of the Aurora B transcript, 5′-GGAAAGAAGGGATCCCTAAdTdT-3′ and Luciferase small interfering RNA, 5′-CTACGCGGAATACTTCGATdTdT-3′. Cell culture and fractionation HeLa cell lines were grown in DMEM containing 10% fetal bovine serum (fetal bovine serum; Hyclone). For the fractionation of cellular extracts, soluble cytoplasmic fractions were lysed with a PA buffer (150 mM Tris–HCl (pH 7.5), 100 mM KCl, 2 mM EDTA, 1 mM PMSF, 1 mM DTT and a mixture of protease inhibitors), whereas supernatants were collected by centrifugation. Insoluble chromatin pellets were washed four times by resuspending them with a wash buffer (100 mM Tris–HCl (pH 7.5), 200 mM KCl, 200 mM EDTA and 250 μM Spermidine trihydrochloride) after mild sonication, and pellets were then collected by centrifugation. Chromatin-bound proteins were obtained by resolubilization into a XBE2 buffer (10 mM HEPES, 2 mM MgCl 2 , 100 mM KCl, 5 mM EGTA and a mixture of protease inhibitors). Cell synchronization For the synchronization experiments described in Fig. 1a,b , Supplementary Fig. 1a,c , HeLa cells were transfected with Lusiferase or Ssu72 small interfering RNA and synchronized in G1/S boundary by double-thymidine block method. Cells were synchronized by the release into fresh media for 3.5 h (S-phase) and 6 h (G2 phase) and labelled with BrdU for 30 min. For the experiments described in Figs 2 , 3 and 4 , HeLa cells were synchronized in the G1/S boundary by using the double-thymidine block, in the S-phase by hydroxy urea treatment (1 mM) for 18 h, in the G2 phase by doxorubicin treatment (150 nM) for 24 h and in mitosis by nocodazole treatment (330 nM) for 16 h. Construction of inducible and stable cell lines For the generation of doxycycline-inducible HeLa cells expressing YFP-Ssu72 WT, S3/4E or S19E fusion proteins, HeLa Tet-on cells were transfected with the pTRE2-hydro vector (BD Biosciences Clontech) containing YFP-fused Ssu72 cDNA sequences. Hygromycin-resistant clones were selected in a culture media containing 400 μg ml −1 hygromycin and induced with 2 μg ml −1 doxycycline for 48 h. The expression of YFP-fused Ssu72 WT, S3/4E or S19E was examined by immunoblotting and immunofluorescence analyses. The HeLa-TAP-Ssu72, HA-tagged Ssu72 (HeLa-HA-Ssu72), and HA-tagged Aurora B (Aur B OE) cell lines were generated by the transfection of HeLa cells with the pIRES puro3 vector (BD Biosciences Clontech) containing the full-length Ssu72 or Aurora B DNA sequence. Puromycin-resistant clones were selected according to the growth in a medium containing 4 μg ml −1 puromycin and were tested in immunoblotting and immunofluorescence assays. The HeLa cells that stably expressed shSsu72 (Ssu72 KD) or shAurora B (Aur B KD) were generated by the transfection of the pSuper puro vector (Oligoengine) containing the Ssu72 shRNA sequence (5′-AAGACCTGTTTGATCTGATCC-3′) or the Aurora B shRNA sequence (5′-CGCGGCACTTCACAATTGATG-3′). Colonies showing resistance to puromycin (2 μg ml −1 ) were selected. Antibodies Rabbit polyclonal antibodies against KLH-conjugated peptides corresponding to phospho-Ser 19 residues (NQNRpSMEAHNILS) of human Ssu72 or to phospho-Ser 1224 residues (MDEpSVLGD) of human SA2 were generated and affinity purified (Young-in Frontier). Mouse monoclonal antibodies to human Ssu72 and rabbit polyclonal antibodies to human SA2 have been described previously [31] . Other antibodies used in this study were obtained as follows: anti-Myc (Roche, Y69 (1:1000) for immunoblotting; (1:300) for immunofluorescence), anti-HA (Roche, 11867431001, 1:1000), anti-phospho-serine (Sigma, P3430, 1:500), anti-phospho-threonine (Cell Signaling, 05–1923, 1:500), anti-Rad21 (Millipore, 05–908, 1:3000), anti-Aurora B (BD Biosciences, 611082 (1:500) for immunoblotting; (1:150) for immunofluorescence), anti-BubR1 (BD Biosciences, 612503, 1:3000), anti-Paxillin (BD Biosciences, 610052, 1:3000), anti-BrdU (Santa Cruz Biotechnology, sc-32323, 1:300 for immunofluorescence), anti-Erk1 (Santa Cruz Biotechnology, sc-93, 1:3000), anti-Erk2 (Santa Cruz Biotechnology, sc-154, 1:3000), anti-histone H3 (Millipore, 05–499, 1:1000), anti-phospho-H3 Ser 10 (Millipore, 05–1336, 1:1000), anti-YFP (Abm, G163, 1:3000), anti-INCENP (Abcam, ab23956, 1:1000), anti-CREST (Immunovision, HCT-0100, 1:1000 for immunofluorescence), anti-Actin (Sigma, A2066, 1:3000), anti-FLAG (Sigma, F7425, 1:3000) and anti-Securin (Zymed, 34–1500, 1:3000). Cell extraction and TAP For immunoprecipitation from total cellular extracts, asynchronized and synchronized cells were resuspended in buffer A (100 mM Tris–HCl (pH 7.5), 20 mM EDTA, 1% NP40, 1 mM PMSF, 1 mM DTT and a protease inhibitor cocktail). The supernatants (soluble cytoplasmic fractions) were obtained, and the remaining cell pellets were resuspended in buffer B (100 mM Tris–HCl (pH 7.5), 20 mM EDTA, 300 mM NaCl, 1.5 mM MgCl 2 , 1% NP40, DNase (2 U μl −1 ) 1 mM PMSF, 1 mM DTT and a protease inhibitor cocktail) and centrifuged and then supernatants (soluble pellet fractions) of pellets were obtained. Mixed extracts (soluble cytoplasmic and pellet supernatants) were diluted with a salt-free buffer solution to reduce the salt concentration to 150 mM. The samples were then centrifuged and analysed by immunoprecipitation. For TAP, HeLa cells expressing TAP-tagged Ssu72 were collected by trypsinization and resuspended in a TNN buffer (50 mM Tris–HCl (pH 7.5), 150 mM NaCl, 1% NP40, 1 mM PMSF, 1 mM DTT and a protease inhibitor cocktail). Beads bound to protein S were incubated with cell extracts (2 mg) for 4 h at 4 °C, washed four times with the TNN buffer and the purified proteins were then used in various assays. GST pull-down assay For the GST pull-down assay, fusion proteins were adsorbed onto glutathione-Sepharose beads (Amersham Biosciences) and incubated with whole-cell extracts (2 mg) from asynchronised HeLa cells for 4 h at 4 °C (ref. 46 ). Bead-bound proteins were separated by SDS–PAGE and then analysed by immunoblotting with appropriate antibodies. In vitro kinase and phosphatase assays For the in vitro kinase assay, purified GST-fused proteins were incubated in a kinase buffer (20 mM HEPES, 1 mM EDTA, 10 mM MgCl2, 100 μM ATP and 5 μCi [γ 32 P]ATP) and 1 μg of the recombinant Aurora B kinase (Sigma) for 1 h at 37 °C. The reaction was stopped by the addition of the SDS sample buffer, resolved by SDS–PAGE, and visualized by autoradiography. For phosphatase analyses, purified GST-Ssu72 WT and MT (GST-Ssu72 S3/4E, GST-Ssu72 S19E, GST-Ssu72 S3/4/19E and GST-Ssu72 C12S) proteins were incubated in a phosphatase buffer containing 10 mM p -nitrophenyl phosphate. The reaction was stopped at the addition of NaOH solution, and phosphatase activity was measured at 405 nm with an ELISA reader. Mass spectrometry For the identification of phosphorylation sites of the human Ssu72 protein during mitosis, TAP-tagged Ssu72 proteins were purified from HeLa-TAP-Ssu72 cells that were incubated in the presence of 200 ng ml −1 nocodazole for 16 h and collected by shake-off. Purified Ssu72 proteins based on agarose beads bound to protein S were resolved with SDS–PAGE and then stained with Coomassie Blue solution. The stained Ssu72 gel band was isolated and washed with 25 mM ammonium bicarbonate, 10 mM DTT and 50 mM iodoacetamide at room temperature for 60 min. The proteins were digested in a solution containing trypsin and elastase proteases at 37 °C for 4 h. Generated peptides were analysed by a LTQ-XL mass spectrometer (Thermo Fisher Scientific) equipped with a nano-LC system (Eksigent) for nano-flow chromatography. Peptides were trapped by a trapping column (internal diameter 75 μm; length=3 cm; particle size=5 μm) and eluted from the column using a mobile-phase gradient onto a reversed-phase analytical column (10 cm × 75 μm internal diameter) packed with C18 (particle size=5 μm). The eluent was then introduced into the LTQ mass spectrometer by a nano-ion source with 1.9 kV of electrospray voltage. Raw data from the LTQ were searched using the IPI human FASTA database (ver. 3.78) with the MASCOT search engine (ver. 2.2.04) selecting the Decoy database analysis. Fluorescence labelling and microscopy For immunostaining, cells were cultured directly on glass coverslips, washed with PBS, fixed in 4% paraformaldehyde and then incubated with the indicated primary and secondary antibodies. For chromosome spreading assays, cells were treated with 100 ng ml −1 colcemid or 200 ng ml −1 nocodazole for 4 h and mitotic cells were collected using the shaking-off method. Mitotic cells (2 × 10 5 ml −1 ) were incubated in a hypotonic buffer (50 mM Tris (pH 7.4) and 55 mM KCl), fixed with freshly made Carnoy’s solution (75% methanol and 25% acetic acid), dropped onto glass slides, and dried at 37 °C. Slides were stained with 5% Giemsa (Merck), washed with PBS, air-dried and processed for fluorescence microscopy. For chromosome-arm-Specific FISH, cells were collected by trypsinization, swollen in a hypotonic buffer (50 mM Tris (pH 7.4) and 55 mM KCl) for 20 m at 37 °C and then fixed twice with Carnoy’s solution (75% methanol and 25% acetic acid) for 15 min. The fixed cells were spun onto glass slides using Shandon Cytospin at 1,500 r.p.m. for 5 min, rehydrated in 2X SSC at 37 °C for 30 min and dehydrated in an ethanol series of 70, 85 and 100% for 2 min each. The samples were denatured in 70% formamide/2 × SSC at 72 °C for 5 min and dehydrated in 70, 85 and 100% ethanol for 2 min each. The samples were hybridized to Cy3-conjugated probes specific to chromosome arm regions (on chromosome 7 and 21), incubated with primary (BrdU) and secondary antibodies (Alexa 568, 1: 300; Molecular Probes) and then stained with DAPI solution. Images were acquired on a LSM510 META confocal microscope fitted with a × 20 NA 0.75 objective lens (Carl Zeiss) and an AxioCam camera (Carl Zeiss). Z series of 0.3 μm stacks were acquired using AxioVision Release 3.x software with Z stack module and deconvolution was performed using Huygens software (Scientific Volume Imaging). The distance between paired FISH signals was measured on the projected images using Huygens software (Scientific Volume Imaging), and the significance of the differences in distance was examined by the statistical Student’s t -test. In vivo ubiquitination assay HeLa cells were transfected with an expression plasmid encoding TAP, TAP-Ssu72 WT, TAP-Ssu72 S19E, Myc-Aurora B or HA-Ubiquitin in combination, as described in Fig. 9 . At 24 h after transfection, the cells from each plate were collected into two aliquots. One aliquot (10%) was used for conventional immunoblotting, and the remaining cells (90%) were used for the purification of TAP-tagged proteins by using agarose beads bound to protein S. The cell lysates were lysed in a TNN buffer and incubated with the agarose beads for 4 h at 4 °C. The beads were washed three times with a TNN buffer and the bound proteins were immunblotted with the indicated antibodies. Analytical gel filtration assay Gel filtration analyses were performed using the Superdex-200 10/300 GL column (Amersham Biosciences). Synchronized HeLa cells were lysed with a TNE buffer (10 mM Tris–HCl (pH 7.5), 200 mM NaCl, 1 mM EDTA, 1 mM PMSF and 1 mM DTT containing a protease inhibitor cocktail) and cleared by ultracentrifugation. The Superdex-200 10/300 GL column (10 mm inter diameter × 300 mm) was equilibrated with a TNE buffer, and cell extracts (500 μl, 20 μg μl −1 ) were then loaded onto the column. Proteins were fractionated with the TNE buffer at a linear flow rate of 0.4 ml min −1 , and 1 ml fractions were collected. How to cite this article: Kim, H.-S. et al. Functional interplay between Aurora B kinase and Ssu72 phosphatase regulates sister chromatid cohesion. Nat. Commun. 4:2631 doi: 10.1038/ncomms3631 (2013).